A Co3O4-CDots-C3N4three component electrocatalyst design concept for efficient and tunable CO2reduction to syngas Syngas, a CO and H 2 mixture mostly generated from non-renewable fossil fuels, is an essential feedstock for production of liquid fuels. Electrochemical reduction of CO 2 and H + /H 2 O is an alternative renewable route to produce syngas. Here we introduce the concept of coupling a hydrogen evolution reaction (HER) catalyst with a CDots/C 3 N 4 composite (a CO 2 reduction catalyst) to achieve a cheap, stable, selective and efficient route for tunable syngas production. Co 3 O 4 , MoS 2 , Au and Pt serve as the HER component. The Co 3 O 4 -CDots-C 3 N 4 electrocatalyst is found to be the most efficient among the combinations studied. The H 2 /CO ratio of the produced syngas is tunable from 0.07:1 to 4:1 by controlling the potential. This catalyst is highly stable for syngas generation (over 100 h) with no other products besides CO and H 2 . Insight into the mechanisms balancing between CO 2 reduction and H 2 evolution when applying the HER-CDots-C 3 N 4 catalyst concept is provided. Syngas, a mixture of H 2 and CO, is a critical feedstock for production of synthetic fuels and industrial chemicals via well-established industrial processes such as the Fischer–Tropsch process (commercialized by Sasol and Shell) [1] , [2] . The H 2 /CO ratio in syngas is of a great significance for meeting the requirements for specific products: H 2 /CO = 2:1 for methanol and H 2 /CO = 1:1 for dimethyl ether for example. The conventional production approach of syngas is based on reforming non-renewable fossil fuels (e.g., coal, petroleum coke, and natural gas) [3] , which increases the consumption of fossil fuel and aggravates the energy crisis. Synthesizing syngas with a controlled H 2 /CO ratio by reduction of CO 2 not only contributes to the solution of the energy crisis, but at the same time reduces the amount of greenhouse gases (CO 2 ). CO 2 reduction to CO and hydrogen evolution reactions (HER) per se are two independent major and important fields. Electrochemical (EC) and photoelectrochemical (PEC) methods integrating CO 2 reduction reaction and HER are key components of prospective technologies for renewable syngas [4] . Different types of semiconductors have been combined with an efficient catalyst for CO 2 reduction to produce syngas by the PEC approach [5] , [6] , [7] , [8] . Cu-ZnO/GaN/n +− p Si was recently reported as a highly efficient PEC catalyst to produce syngas with a tunable H 2 /CO ratio (between 1:2 and 4:1) [5] . Metal or metal-based composites, including Ag [9] , Cu [10] , Ru(II) polypyridyl complex [11] , Ag/C 3 N 4 [12] , and Re-functionalized graphene oxide [13] , have been investigated for EC reduction of CO 2 and H + /H 2 O to syngas. The different methods used to tune the ratio of H 2 /CO include altering the CO 2 flow rate [14] and pressure [15] , the reaction temperature [16] , and the applied potential [9] . Different crystalline sites of Au catalyze different reaction channels (edge sites initiate CO generation and corner sites H 2 generation) [17] , [18] . A novel pulsed-bias technique using Cu as the catalyst was recently applied to tune the H 2 /CO ratio in syngas between ~32:1 and 9:16 by using different pulse times for the same working potential. The selectivity is however limited and CH 4 and C 2 H 4 by-products affect the purity of syngas [10] . Using Ag/C 3 N 4 [12] , the H 2 /CO ratio in the produced syngas can be tuned from 100:1 to 2:1 by controlling the applied potential and the Ag loading on graphitic carbon nitride but the total current density is lower than 1 mA/cm 2 at −0.6 V. The previous EC attempts to synthesize renewable syngas are still characterized by an unsatisfactory performance including some of the following disadvantages: a high onset overpotential necessary to initiate the CO 2 reduction reaction, a low CO + H 2 generation current density, a small selectivity of CO production, and a poor stability of the generation current density and the Faradaic efficiency (FE) of H 2 and CO. We hereby propose a design concept of a cheap composite EC catalyst for a tunable, stable, selective, and efficient production of syngas, made of three components: a HER catalyst, a CO 2 reduction catalyst toward CO, and a catalyst which stabilizes the active hydrogen (H•) necessary to trigger both HER and the CO 2 reduction reactions. For HER, we choose several known catalysts (Co 3 O 4 , Pt, MoS 2 , and Au). For CO 2 reduction, we apply graphitic carbon nitride (C 3 N 4 ) since carbon-bonded nitrogen groups including pyridinic N, pyrrolic N, and graphitic N have recently been proposed as active sites for CO 2 reduction to CO [19] , [20] , [21] . C 3 N 4 has a porous structure and is shown as a good substrate for dispersion of catalytic nanoparticles [22] , [23] , [24] , [25] . The selected catalyst for stabilization of active hydrogen (H•) are carbon dots (CDots) [26] , [27] , which possess significant adsorption capabilities for H + [28] , [29] and CO 2 [30] and exhibit excellent ability of electron transfer [31] , [32] necessary for H• generation (H + +e − →H•). CDots also improve the conductivity of C 3 N 4 . Here we found that the Co 3 O 4 -CDots-C 3 N 4 is the best EC catalyst for syngas production studied within the present work. We thus first describe the structural characterization of this catalyst. We then present the design concept of the three-component catalyst for syngas production and detail its working mechanisms. We follow by showing that this concept is valid and that Co 3 O 4 -CDots-C 3 N 4 is indeed an efficient, tunable, stable, selective, and cheap EC catalyst for syngas production. It initiates CO 2 reduction to CO in aqueous solutions at a low overpotential (0.17 V vs. reversible hydrogen electrode (RHE)) and the total current density of H 2 and CO generation may reach up to 15 mA/cm 2 at a potential of −1.0 V vs. RHE. The H 2 /CO ratio of syngas generated by Co 3 O 4 -CDots-C 3 N 4 is tunable from 0.07:1 to 4:1 by controlling the applied potential. Dedicated experiments highlight the different mechanisms by which syngas production applying Co 3 O 4 -CDots-C 3 N 4 is controlled and manipulated. Finally, the generality of the catalyst design concept applying Pt, MoS 2 , and Au as the HER catalyst is demonstrated. The significance of this work is thus twofold. First, it presents Co 3 O 4 -CDots-C 3 N 4 as an efficient, cheap, tunable, and stable catalyst for syngas production on one hand. Second, it provides an avenue to design catalysts for controlled and tuned production of syngas in particular and other chemicals of interest to the chemical industry in general. Characterization of Co 3 O 4 -CDots-C 3 N 4 Transmission electron microscopy (TEM) image (Fig. 1a ) reveals that the Co 3 O 4 -CDots-C 3 N 4 consist of nm-sized Co 3 O 4 nanoparticles (NPs) and CDots dispersed on the C 3 N 4 matrix. The two different types of nanocrystals shown in the inset of Fig. 1a are identified as Co 3 O 4 NPs with a d-spacing of 0.24 nm consistent with Co 3 O 4 (311) [33] and CDots with an interplanar spacing of 0.33 nm (see Supplementary Fig. 1 ) [34] . 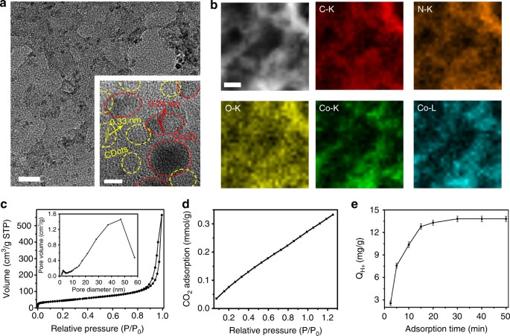Fig. 1 Characterization of the Co3O4-CDots-C3N4.aTEM image of a grain of the Co3O4-CDots-C3N4and a HRTEM image of Co3O4-CDots-C3N4(inset), scale bar 20 nm and 5 nm (inset).bSTEM micrograph and the corresponding elemental mapping of C-K, N-K, O-K, Co-K, and Co-L for the Co3O4-CDots-C3N4, scale bar 50 nm.cN2adsorption–desorption isotherm and the corresponding pore-size distribution of Co3O4-CDots-C3N4(inset).dCO2adsorption isotherm of Co3O4-CDots-C3N4.eThe time-course adsorption of H+by the Co3O4-CDots-C3N4. The adsorption is 13.8 mg/g. Experiments were performed in triplicates and results are shown as mean ± standard deviation Figure 1b displays a scanning transmission electron microscopy (STEM) micrograph and its corresponding chemical maps of C-K, N-K, O-K, Co-K, and Co-L for the Co 3 O 4 -CDots-C 3 N 4 . Co-K, Co-L, and O-K cover the entire C 3 N 4 area monitored, indicating that Co 3 O 4 NPs are evenly distributed on the C 3 N 4 sheet. X-ray diffraction (XRD) shows (Supplementary Fig. 2 ) the typical diffraction lines of Co 3 O 4 and C 3 N 4 . Besides the average size of Co 3 O 4 NPs derived from the XRD spectrum of the Co 3 O 4 -CDots-C 3 N 4 using the Debye−Scherrer equation (Supplementary Table 1 ), is about 10 nm, which is consistent with the size of Co 3 O 4 NPs in the TEM image. Energy dispersive X-ray absorption (EDX) analysis of the Co 3 O 4 -CDots-C 3 N 4 (Supplementary Fig. 3 ) reveals an elemental atom composition of C (46.65 at. %), N (48.74 at. %), O (3.01 at. %), and Co (1.60 at. %). X-ray photoelectron spectroscopy (XPS) of the composite (Supplementary Fig. 4 ) shows C 1s, N 1s, O 1s, and Co 2p peaks with a similar elemental composition to that deduced by EDX (C (39.9 at. %), N (52.5 at. %), O (5.8 at. %), and Co (1.8 at. 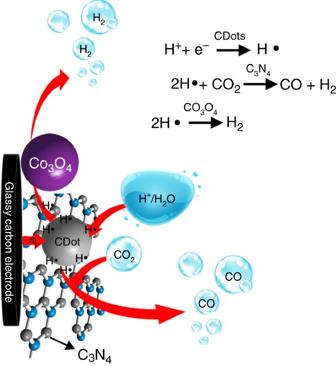Fig. 2 Schematic diagram of the reaction mechanism induced by Co3O4-CDots-C3N4. CDots are the generation site of H•, Co3O4the generation site of H2, and C3N4the generation site of CO %)) (Supplementary Table 2 ). The Co 2p 3/2 peak was fitted (Supplementary Fig. 4e ) by using two synthetic peaks positioned at binding energy (BE) = 780.0 and 781.3 eV (Co 3+ and Co 2+ , respectively) and the Co 2p 1/2 peak was fitted (Supplementary Fig. 4e ) by using two synthetic peaks positioned at BE = 795.0 and 797.3 eV (Co 3+ and Co 2+ , respectively). Figure 1c shows type IV N 2 adsorption–desorption isotherms of the Co 3 O 4 -CDots-C 3 N 4 with a H3-type hysteresis loop [35] , indicating the formation of a porous structure (the pore-size distribution was derived from the isotherms; for more details, see Supplementary Methods ) is presented in Fig. 1c inset; specific surface area ~160 m 2 /g). The porous Co 3 O 4 -CDots-C 3 N 4 was found to adsorb a large amount of CO 2 (~0.33 mmol/g at 1.2 atm, Fig. 1d ). This strong CO 2 adsorption capability is mainly due to CO 2 molecules adsorbed on the porous C 3 N 4 surfaces, which constitute more than 90 wt.% of the composite catalyst (Supplementary Fig. 5a ). It is nevertheless enhanced in a synergistic way by the incorporation of CDots (Supplementary Fig. 5b shows that the CO 2 adsorption on Co 3 O 4 -CDots-C 3 N 4 and on CDots-C 3 N 4 is about the same, while that on Co 3 O 4 -C 3 N 4 is much lower). The adsorption of H + (Fig. 1e ) is very rapid in the first 15 min, then it becomes slower with contact time, stopping additional absorption after 30 min. The amount of adsorbed H + (for more details, see Supplementary Methods ) on Co 3 O 4 -CDots-C 3 N 4 and CDots-C 3 N 4 is about 13.8 mg/g, while the amount of adsorbed H + is only 5.11 mg/g for the Co 3 O 4 -C 3 N 4 (Supplementary Fig. 6b ). The incorporation of CDots thus significantly increases the adsorbed capacity of H + . All these results indicate that the present electrocatalyst has a strong adsorption capacity for both H + and CO 2 , which is significantly important for both processes of CO 2 reduction reaction and HER. Fig. 1 Characterization of the Co 3 O 4 -CDots-C 3 N 4 . a TEM image of a grain of the Co 3 O 4 -CDots-C 3 N 4 and a HRTEM image of Co 3 O 4 -CDots-C 3 N 4 (inset), scale bar 20 nm and 5 nm (inset). b STEM micrograph and the corresponding elemental mapping of C-K, N-K, O-K, Co-K, and Co-L for the Co 3 O 4 -CDots-C 3 N 4 , scale bar 50 nm. c N 2 adsorption–desorption isotherm and the corresponding pore-size distribution of Co 3 O 4 -CDots-C 3 N 4 (inset). d CO 2 adsorption isotherm of Co 3 O 4 -CDots-C 3 N 4 . e The time-course adsorption of H + by the Co 3 O 4 -CDots-C 3 N 4 . The adsorption is 13.8 mg/g. Experiments were performed in triplicates and results are shown as mean ± standard deviation Full size image The electrocatalyst design and reaction mechanism We first present the design concept of the ternary electrocatalyst and highlight its operation mode to produce syngas in a controllable, tunable way. The proposed electrocatalyst consists of three parts: an electrocatalyst for HER (e.g., Co 3 O 4 ), an electrocatalyst for CO 2 reduction to CO (e.g., C 3 N 4 ), and an electrocatalyst which triggers both reaction channels (e.g., CDots by trapping H + and e − and generating H•). A schematic diagram of the Co 3 O 4 -CDots-C 3 N 4 ternary electrocatalyst syngas generation is presented in Fig. 2 . CDots first trap H + from the solution and e − from the glassy carbon electrodes and combine them to form H•. The two other catalyst components compete for these H• species. They may diffuse to C 3 N 4 (the CO 2 reduction catalyst due to its different N active sites [19] , [20] , [21] ) and reduce CO 2 to CO. Alternatively they may diffuse to Co 3 O 4 (the HER catalyst) and produce H 2 . We thus suggest that CDots are the generation site of H•, C 3 N 4 is the generation site of CO, and Co 3 O 4 is the generation site of H 2 . Syngas with tunable H 2 /CO ratio can be thus achieved by balancing the CO 2 reduction channel and the HER channel. The different catalyst components have additional functions. Introduction of CDots to the composites enhances the adsorption of both CO 2 and H + . Incorporation of CDots in the electrocatalyst improves its conductivity (Supplementary Fig. 7 ). C 3 N 4 serves as the highly porous substrate in which the CDots and Co 3 O 4 nanoparticles are incorporated. C 3 N 4 thus provides a large surface area which enhances the reaction activity and also guarantees a proximity between the different generation sites (CDots for H• generation, C 3 N 4 for CO generation, and Co 3 O 4 for H 2 generation). This proximity is essential for an efficient reaction. Experimental evidence substantiating this proposed mechanism will be given in the following sections. Fig. 2 Schematic diagram of the reaction mechanism induced by Co 3 O 4 -CDots-C 3 N 4 . CDots are the generation site of H•, Co 3 O 4 the generation site of H 2 , and C 3 N 4 the generation site of CO Full size image The electrocatalytic performance of Co 3 O 4 -CDots-C 3 N 4 We now show that the suggested design concept of the Co 3 O 4 -CDots-C 3 N 4 indeed provides a tunable and stable production of syngas. The electrocatalytic performance of Co 3 O 4 -CDots-C 3 N 4 for syngas production was tested in an airtight three electrodes electrochemical H-type cell. The gaseous reduction products monitored by a gas chromatography (GC) system were CO and H 2 while no other reduction liquid products were found by H 1 NMR. 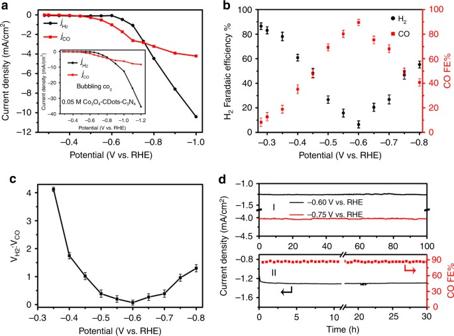Fig. 3 Electroreduction of CO2and H+/H2O to syngas with adjustable H2/CO ratio.aThe current density for HER (jH2, black trace) and for CO2reduction, (jCO, red trace) vs. the applied potential, catalyzed by Co3O4-CDots-C3N4in CO2-saturated 0.5 M KHCO3electrolyte. The inset shows the same experiment conducted with bubbling of CO2to the solution to overcome CO2consumption during the experiment.bThe FEs of the reduction of CO2to CO (red points) and H+to H2(black points) catalyzed by Co3O4-CDots-C3N4vs. the applied potential. Experiments were performed in triplicates and results are shown as mean ± standard deviation.cThe volume ratio between H2and CO vs. the applied potential. The H2/CO volume ratio is about 1:1 at the potential of −0.45 V or −0.75 V vs. RHE.dThe stability of the performance of Co3O4-CDots-C3N4for producing syngas: operated at potentiostatic potential of −0.6 and −0.75 V for 100 h (dΙ); operated at potentiostatic potential of −0.6 V for 30 h (dII): current density vs. time (left axis) and FEs of CO production vs. time (right axis) Figure 3a shows the current densities of CO ( j CO , red trace) and H 2 ( j H2 , black trace) vs. different potentials acquired in a CO 2 -saturated 0.5 M KHCO 3 (pH = 7.2) solution. The curves indicate a significant generation of both CO and H 2 but the j CO / j H2 ratio varies with the potential applied. The j CO curve shows that the CO 2 electrocatalytic reduction starts at an initial potential of −0.28 V vs. RHE (all potentials reported throughout this paper are with respect to this reference). This operating voltage corresponds to a low overpotential of 0.17 V (the equilibrium potential of CO 2 /CO is at −0.11 V). Up to −0.45 V, both j CO and j H2 are very small and above −0.45 V both currents increase. Between −0.45 and −0.75 V, j CO is larger than j H2 , indicating that the CO 2 reduction reaction predominates. For potentials larger than −0.75 V, the HER channel becomes more significant than the CO 2 reduction reaction. The increase of j H2 with potential is about constant (the j H2 curve is a straight line). In contrast, the slope of the j CO curve decreases with the potential applied. We attribute this behavior to the consumption of CO 2 at high CO generation rates due to its low solubility or slow mass transfer. Indeed (inset of Fig. 3a ), bubbling CO 2 into the electrolyte increases j CO but the increase rate of j CO with potential is still lower than that of j H2 . Figure 3b shows the FEs of CO and H 2 generation vs. the applied cathodic potentials. The FE of CO generation increases with the applied potential and reaches a maximum of 89% at −0.6 V. For higher potential, it decreases to ~40% with increasing potential to −0.8 V, most probably due to the limited mass transport of CO 2 in the electrolyte. In contrast, the FE of H 2 generation is about 86% for a low applied potential, decreases with potential to about 5% at −0.6 V and then rises again reaching 55% at −0.8 V. The total FE of CO and H 2 combined reaches up to 95%. Consequently, syngas with different H 2 /CO ratios can be obtained by altering the applied potential as shown in Fig. 3c . The volume ratio between H 2 and CO can be tuned from 4:1 to 0.07:1 and syngas with H 2 /CO = 1:1 can directly be generated at the potentials of −0.45 V (total current density is 0.25 mA/cm 2 ) and −0.75 V (total current density is 5.78 mA/cm 2 ). Note that the catalyst mass activity for syngas generation reaches a high value of 10 A/g catalyst at a potential of −0.6 V. The stability of the Co 3 O 4 -CDots-C 3 N 4 catalyst for electrocatalytic CO 2 reduction and HER (Fig. 3d ) was studied as well. A negligible decay in current density was observed when operating the system for 100 h at the applied potential of both −0.6 V (Fig. 3dΙ , black trace, CO 2 reduction reaction predominates) and −0.75 V (Fig. 3dΙ , red trace, HER and CO 2 reduction are equal). It reveals that the Co 3 O 4 -CDots-C 3 N 4 maintains high electrocatalytic stability during the 100-h test. An additional experiment validated the stability of both the current density and the FE for 30 h (it is very likely that the FE is stable for 100 h as well). Fig. 3 Electroreduction of CO 2 and H + /H 2 O to syngas with adjustable H 2 /CO ratio. a The current density for HER ( j H2 , black trace) and for CO 2 reduction, ( j CO , red trace) vs. the applied potential, catalyzed by Co 3 O 4 -CDots-C 3 N 4 in CO 2 -saturated 0.5 M KHCO 3 electrolyte. The inset shows the same experiment conducted with bubbling of CO 2 to the solution to overcome CO 2 consumption during the experiment. b The FEs of the reduction of CO 2 to CO (red points) and H + to H 2 (black points) catalyzed by Co 3 O 4 -CDots-C 3 N 4 vs. the applied potential. Experiments were performed in triplicates and results are shown as mean ± standard deviation. c The volume ratio between H 2 and CO vs. the applied potential. The H 2 /CO volume ratio is about 1:1 at the potential of −0.45 V or −0.75 V vs. RHE. d The stability of the performance of Co 3 O 4 -CDots-C 3 N 4 for producing syngas: operated at potentiostatic potential of −0.6 and −0.75 V for 100 h ( dΙ ); operated at potentiostatic potential of −0.6 V for 30 h ( dII ): current density vs. time (left axis) and FEs of CO production vs. time (right axis) Full size image Investigation of the catalytic mechanisms A series of controlled experiments were carried out to validate and further understand the catalytic mechanism operating with the Co 3 O 4 -CDots-C 3 N 4 proposed in a previous section (Fig. 2 ). Issues investigated included: the generation sites of H•, CO, and H 2 ; the role of H + ; the roles of CDots, C 3 N 4 , and Co 3 O 4 ; the role of the proximity between the CDots, C 3 N 4 , and Co 3 O 4 ; ways in which the relative significance of the different reaction channels and the resulting CO/H 2 volume ratio can be manipulated; other HER-CDots-C 3 N 4 systems with different HER materials. We first studied the linear sweep voltammetry (LSV) curves of different combinations of the three components comprising the ternary Co 3 O 4 -CDots-C 3 N 4 . The comparison of the different LSV curves (Fig. 4a ) and the complementary study of the CO and H 2 composition generated during the electrocatalytic processes catalyzed by the different components (Fig. 4b ) enabled a clear determination of both the generation sites of the CO and H 2 and the role of the three basic components used. We first discuss the LSVs showing the apparent current density (current density per geometrical area), which is also equivalent to the mass activity of the catalysts (current per gram catalyst) as shown in Fig. 4a . Further on, we also give the corresponding turn on frequencies (TOFs) and the real current densities derived from the real surface areas of the components of the different combinations of catalysts in Fig. 4a . LSVs of C 3 N 4 (Fig. 4a , curve 1, black trace, morphology of C 3 N 4 is shown in Supplementary Fig. 8a ), CDots (Fig. 4a , curve 2, cyan trace, morphology of CDots is shown in Supplementary Fig. 1 ), Co 3 O 4 (curve 3, gray trace, morphology of Co 3 O 4 is shown in Supplementary Fig. 8b ), CDots-C 3 N 4 (curve 4, blue trace, morphology of CDots-C 3 N 4 is shown in Supplementary Fig. 8c ), Co 3 O 4 -C 3 N 4 (curve 5, green trace, morphology of Co 3 O 4 -C 3 N 4 is shown in Supplementary Fig. 8d ), Co 3 O 4 -CDots (curve 6, purple trace, morphology of Co 3 O 4 -CDots is shown in Supplementary Fig. 8e ), and Co 3 O 4 -CDots-C 3 N 4 (curve 7, red trace) were performed using a CO 2 -saturated 0.5 M KHCO 3 (pH = 7.2) solution (Fig. 4a ). The LSVs of C 3 N 4 (curve 1, black trace), CDots (curve 2, cyan trace), Co 3 O 4 (curve 3, gray trace), CDots-C 3 N 4 (curve 4, blue trace), and Co 3 O 4 -C 3 N 4 (curve 5, green trace) show poor electrocatalytic performances evident by their low current densities and high onset potentials (Fig. 4a ). Only the Co 3 O 4 -CDots (curve 6) and the Co 3 O 4 -CDots-C 3 N 4 (curve 7) exhibit high current densities and low onset potentials (Fig. 4a ). CDots generate H 2 only, but not CO (Fig. 4b ). We explain it by their trapping and stabilizing H•, which may generate a small amount of H 2 even in the absence of a HER catalyst. The LSV of Co 3 O 4 (curve 3, gray trace) shows a relatively small activity producing only H 2 (Fig. 4b ). In comparison, Co 3 O 4 -CDots (curve 6, purple trace) produces a much larger amount of H 2 compared to pure CDots or pure Co 3 O 4 . We attribute it to the effect of the CDots, which greatly enhance the electrocatalytic performance of Co 3 O 4 by providing H•, which is necessary for generation of H 2 . We thus conclude that Co 3 O 4 is the H 2 generation site while CDots are the generation site of H• and both are needed for a large generation rate of H 2 . Now, we prove that the generation site of CO is C 3 N 4 . Figures 3 a, b and 4a, b indicate that significant amounts of CO are generated by either the CDots-C 3 N 4 or the Co 3 O 4 -CDots-C 3 N 4 . Co 3 O 4 was shown to generate H 2 only, which leaves CDots-C 3 N 4 as the producer of CO. CDots per se produce only H 2 as previously discussed. They however are essential for CO generation by CDots-C 3 N 4 since they significantly enhance the CO 2 adsorption, adsorb H + , and stabilize H•. C 3 N 4 per se catalyzes only a very small (negligible) current (Fig. 4a , curve 1) so that the very little amount of gas produced by pure C 3 N 4 (Fig. 4b ) contains more H 2 than CO. The supply of H• by the CDots is necessary to promote the generation of CO in C 3 N 4 . 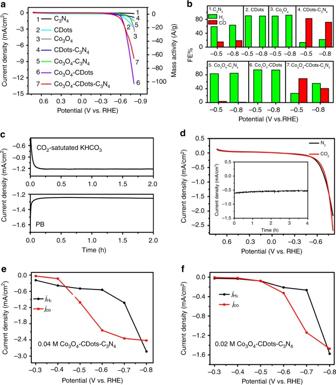Fig. 4 Electrochemical experiments providing insight into the electrochemical processes.aThe linear sweep voltammetry curves (LSVs) for C3N4(black trace, curve 1), CDots (cyan trace, curve 2), Co3O4(gray trace, curve 3), CDots-C3N4(blue trace, curve 4), Co3O4-C3N4(green trace, curve 5), Co3O4-CDots (purple trace, curve 6), and Co3O4-CDots-C3N4(red trace, curve 7) in CO2-saturated 0.5 M KHCO3electrolyte, 10 mV/s. Current density on leftyaxis and mass activity on rightyaxis. The comparison of the curves allows determination of the role of the different catalyst components in the electrochemical reactions.bThe FEs of the reaction products at −0.5 and −0.8 V, using C3N4, CDots, Co3O4, CDots-C3N4, Co3O4-C3N4, Co3O4-CDots, and Co3O4-CDots-C3N4, respectively, as catalysts. Note that only the C3N4and CDots-C3N4composites produce significant amounts of CO.cTotal current density vs. time curves of CO2reduction to CO and HER at the potential of −0.6 V in CO2-saturated KHCO3solution (0.5 M, pH = 7.2) and phosphate buffer (PB) solution (pH = 7.2), respectively.dLSVs for the Co3O4-CDots-C3N4in N2- (black trace) and CO2-saturated (red trace) MeCN containing 0.5 M [BMIM]PF6, 10 mV/s. The inset shows the total current density vs. time curves of CO2reduction at the potential of −0.6 V in CO2-saturated MeCN containing 0.5 M [BMIM]PF6. The current in the inset is much smaller than incand no reaction products are detected indicating that H+is essential for both HER and CO2reduction to CO.eCurrent density for HER (jH2, black trace) and current density for CO2reduction, (jCO, red trace) vs. the applied potential, catalyzed by 0.04 M Co3O4-CDots-C3N4in a CO2-saturated 0.5 M KHCO3electrolyte.fCurrent density for HER (jH2, black trace) and current density for CO2reduction, (jCO, red trace) vs. the applied potential, catalyzed by 0.02 M Co3O4-CDots-C3N4in CO2-saturated 0.5 M KHCO3electrolyte; note that the reduction of the amount of the HER catalyst component shifts the balance of gas generation toward enhanced CO generation 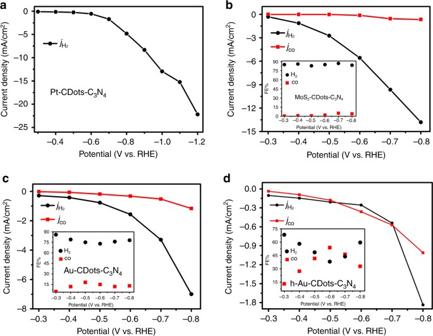Fig. 5 Catalytic activity of composite catalysts with different HER catalysts.aCurrent density for HER (jH2, black trace) vs. the applied potential, catalyzed by Pt-CDots-C3N4in CO2-saturated 0.5 M KHCO3electrolyte.bCurrent density for HER (jH2, black trace) and current density for CO2reduction to CO, (jco, red trace) and FEs of H2and CO (inset) vs. the applied potential, catalyzed by MoS2-CDots-C3N4in CO2-saturated 0.5 M KHCO3electrolyte.cCurrent density for HER (jH2, black trace) and current density for CO2reduction, (jco, red trace) and FEs of H2and CO (inset) vs. the applied potential, catalyzed by Au-CDots-C3N4in CO2-saturated 0.5 M KHCO3electrolyte.dCurrent density for HER (jH2, black trace) and current density for CO2reduction, (jco, red trace) and FEs of H2and CO (inset) vs. the applied potential, catalyzed by Au-CDots-C3N4in CO2-saturated 0.5 M KHCO3electrolyte. The amount of Au indis half of that inc(marked as h-Au-CDots-C3N4) leading to an increase of the CO/H2ratio indwith respect to that inc Figure 4a shows that each catalyst component adds to the activity by enhancing one of the three reactions (H• generation, H 2 generation, and CO generation) but the complete three components composite Co 3 O 4 -CDots-C 3 N 4 is necessary for intense generation of syngas. We further studied the effect of the type of mixing of the different catalyst components on the catalytic activity. The LSVs of physical mixtures of catalysts (Co 3 O 4 + C 3 N 4 , CDots + C 3 N 4 , and Co 3 O 4 + CDots + C 3 N 4 ) were compared to those of composites of the same components chemically blended (Co 3 O 4 -C 3 N 4 , CDots-C 3 N 4 , and Co 3 O 4 -CDots-C 3 N 4 ). The chemically prepared composites had much larger activities (current densities) than their corresponding physical mixtures (Supplementary Fig. 9 ). We attribute the large activity of the chemically prepared composites to the close proximity between the different catalysts (active sites) in the composite materials. In contrast, physical mixing does not provide such a proximity so that the large distance between the active sites hinders the activity of the physically mixed catalysts. Fig. 4 Electrochemical experiments providing insight into the electrochemical processes. a The linear sweep voltammetry curves (LSVs) for C 3 N 4 (black trace, curve 1), CDots (cyan trace, curve 2), Co 3 O 4 (gray trace, curve 3), CDots-C 3 N 4 (blue trace, curve 4), Co 3 O 4 -C 3 N 4 (green trace, curve 5), Co 3 O 4 -CDots (purple trace, curve 6), and Co 3 O 4 -CDots-C 3 N 4 (red trace, curve 7) in CO 2 -saturated 0.5 M KHCO 3 electrolyte, 10 mV/s. Current density on left y axis and mass activity on right y axis. The comparison of the curves allows determination of the role of the different catalyst components in the electrochemical reactions. b The FEs of the reaction products at −0.5 and −0.8 V, using C 3 N 4 , CDots, Co 3 O 4 , CDots-C 3 N 4 , Co 3 O 4 -C 3 N 4 , Co 3 O 4 -CDots, and Co 3 O 4 -CDots-C 3 N 4 , respectively, as catalysts. Note that only the C 3 N 4 and CDots-C 3 N 4 composites produce significant amounts of CO. c Total current density vs. time curves of CO 2 reduction to CO and HER at the potential of −0.6 V in CO 2 -saturated KHCO 3 solution (0.5 M, pH = 7.2) and phosphate buffer (PB) solution (pH = 7.2), respectively. d LSVs for the Co 3 O 4 -CDots-C 3 N 4 in N 2 - (black trace) and CO 2 -saturated (red trace) MeCN containing 0.5 M [BMIM]PF 6 , 10 mV/s. The inset shows the total current density vs. time curves of CO 2 reduction at the potential of −0.6 V in CO 2 -saturated MeCN containing 0.5 M [BMIM]PF 6 . The current in the inset is much smaller than in c and no reaction products are detected indicating that H + is essential for both HER and CO 2 reduction to CO. e Current density for HER ( j H2 , black trace) and current density for CO 2 reduction, ( j CO , red trace) vs. the applied potential, catalyzed by 0.04 M Co 3 O 4 -CDots-C 3 N 4 in a CO 2 -saturated 0.5 M KHCO 3 electrolyte. f Current density for HER ( j H2 , black trace) and current density for CO 2 reduction, ( j CO , red trace) vs. the applied potential, catalyzed by 0.02 M Co 3 O 4 -CDots-C 3 N 4 in CO 2 -saturated 0.5 M KHCO 3 electrolyte; note that the reduction of the amount of the HER catalyst component shifts the balance of gas generation toward enhanced CO generation Full size image The comparison between the LSVs of the different catalyst components and their composites (Fig. 4a ) should be done carefully. The catalyst areal density was kept the same (0.127 mg/cm 2 ) for all (3 mm in diameter) electrodes. Since the composition of the Co 3 O 4 -CDots-C 3 N 4 was 6 wt% Co 3 O 4 , 1 wt% CDots, and 93 wt% C 3 N 4 , it follows that the amount of CDots or Co 3 O 4 in the CDots, Co 3 O 4 , or Co 3 O 4 -CDots electrodes was much larger than in the C 3 N 4 containing composite electrodes. This means that the reaction activity per catalyst mass of curves 2, 3, and 6 is very low compared to that of the Co 3 O 4 -CDots-C 3 N 4 electrode (Fig. 4a , curve 7). Since we deal with three different catalysts with different functions, we should calculate the mass activity (current per gram catalyst) for each component separately. This was done in Supplementary Fig. 10 . The reaction activity per mass of a single catalyst component (Co 3 O 4 or CDots) of Co 3 O 4 -CDots (Fig. 4a , curve 6), e.g., is actually lower by more than an order of magnitude than the activity per mass of a single catalyst component of that of the Co 3 O 4 -CDots-C 3 N 4 catalyst (Fig. 4a , curve 7) though curve 6 appears to indicate (Fig. 4a ) a larger activity than curve 7 (compare Fig. 4a to Supplementary Fig. 10 ). Supplementary Fig. 10 clearly shows that starting from a single catalyst component, the addition of each of the two other components increases the activity of syngas production, i.e., all components are necessary for an optimized syngas generation. Similarly, we calculate the turn on frequencies (TOFs) of the catalysts compositions of Fig. 4a . TOF = (number of reacted electrons per time/number of catalyst active sites). We approximate the number of active sites by the number of catalyst atoms. Since we have three different catalyst components with three different functions, we calculate the TOFs per each catalyst component (CDots, Co 3 O 4 , and C 3 N 4 ). Supplementary Fig. 11 shows (similar to Supplementary Fig. 10 ) that the addition of each single component increases the syngas production activity and all components are necessary for the optimal performance. We further measure the BET and the electrochemical real surface areas of the catalyst components of each combination shown in curves 1–7 (Supplementary Tables 3 – 4 ). We use the electrochemical surface areas (ECSAs) to calculate the real current densities related to the specific catalyst components that constitute the seven combinations shown in curves 1–7. Supplementary Fig. 12 shows that similar to the mass activities and the TOFs curves, the real current densities of one component increase with the addition of a second component and are the largest when all three catalyst components combine to a three-component catalyst composite. Figure 3 shows that the ternary concept design indeed yields an optimal performance of its different components balancing between CO 2 reduction and HER. This explains the high value of 10 A/g catalyst obtained at −0.6 V. The CO 2 and H + adsorption measurements (Supplementary Figs. 5 and 6 ) of the individual different catalyst components (CDots, Co 3 O 4 , and C 3 N 4 ) and their composites (CDots-C 3 N 4 , Co 3 O 4 -C 3 N 4 , CDots-Co 3 O 4 , and CO 3 O 4 -CDots-C 3 N 4 ) reveal another effect which improves the ternary composite catalyst performance. The synergism of the three components acting simultaneously enhances the adsorption of the ternary composite by a factor of 2–3 with respect to the adsorption of the individual components. Real surface area measurements (BET and electrochemical) of the catalyst compositions (Supplementary Table 3 ) indicate that the inclusion of the C 3 N 4 component results in a high surface area ((S real /S geometrical ) = 200 for BET and 30 for electrochemical) while it is lower by an order of magnitude for the nanoparticle catalysts (CDots, Co 3 O 4 , or CDots-Co 3 O 4 ). The dispersion of the catalysts nanoparticles on the C 3 N 4 surface seems to explain the synergistic adsorption behavior. To study the role of H + in syngas generation, we investigated the electrocatalytic performance of Co 3 O 4 -CDots-C 3 N 4 in aqueous solutions with the same pH value (HER in phosphate buffer solution, pH = 7.2; syngas reaction in CO 2 -saturated 0.5 M KHCO 3 solution, pH = 7.2) and in an ionic liquid (without H + ). The current density–time curves of pure HER and syngas reactions at the potential of −0.6 V (at −0.6 V the syngas reaction produces ~90% CO) are shown in Fig. 4c . A stable current density (~−1.21 mA/cm 2 ) for syngas is observed at −0.6 V while −1.25 mA/cm 2 for HER is reached at the same potential. Then, ionic liquid was used as the electrolyte solution to eliminate H + . The electrocatalytic performance of Co 3 O 4 -CDots-C 3 N 4 was tested at the potential of −0.6 V in a CO 2 -saturated MeCN solution containing 0.5 M [BMIM]PF 6 . The current density is only about 0.61 mA/cm 2 in a CO 2 -saturated ionic liquid (Fig. 4d ), which is much lower than that obtained for CO 2 reduction in CO 2 -saturated KHCO 3 solution (−1.21 mA/cm 2 ). Notably, no gaseous products of CO reduction could be detected suggesting that H + plays an important role for CO 2 reduction to CO in the present Co 3 O 4 -CDots-C 3 N 4 catalyst system. It was shown that the H 2 /CO volume ratio obtained using the Co 3 O 4 -CDots-C 3 N 4 catalyst system is determined by the balance between the HER channel and the CO 2 reduction channel to CO. This ratio was tuned by modifying the potential (Fig. 3 ). Another plausible tuning method is the decrease of the amount of the HER catalyst component (Co 3 O 4 ) thus reducing the HER activity and increasing the CO 2 reduction activity. We therefore measured the electrocatalytic activities of Co 3 O 4 -CDots-C 3 N 4 produced using lower amounts of Co (0.04 and 0.02 M Co 3 O 4 loadings with respect to the standard one of the present work (0.05 M)). Figures 3 a and 4e, f show the j H2 and j CO obtained at different applied potentials for 0.05, 0.04, and 0.02 M Co 3 O 4 -CDots-C 3 N 4 , respectively. It is obvious that the CO/H 2 ratio was strongly affected by the change of the Co 3 O 4 HER catalyst amount. Finally, the design concept of the HER-CDots-C 3 N 4 ternary catalyst was applied for three additional HER active electrocatalysts: Pt, MoS 2 , and Au to form Pt-CDots-C 3 N 4 , MoS 2 -CDots-C 3 N 4 , and Au-CDots-C 3 N 4 . The structural characterization of these catalysts is given in Supplementary Fig. 13 . The electrocatalytic activity of these three ternary composite catalysts for producing syngas were tested under the same conditions as for Co 3 O 4 -CDots-C 3 N 4 . Applying the Pt-CDots-C 3 N 4 electrocatalyst (Fig. 5a ), only hydrogen was detected in the gas phase and no reduction products from CO 2 reduction were observed. Pt is considered as the most efficient electrocatalyst to facilitate HER [36] . The application of Pt-CDots-C 3 N 4 as a catalyst shifts the balance between HER and CO 2 reduction toward H 2 generation, increases the intensity of the efficient HER channel and completely suppresses the CO 2 reduction to CO. The MoS 2 -CDots-C 3 N 4 electrocatalyst is still sufficiently HER active to produce close to 90% j H2 , but a small amount of j CO (a few percent of the total current) is nevertheless observed. The FEs of CO are no more than 10% for the MoS 2 -CDots-C 3 N 4 (inset of Fig. 5b ). The Au-CDots-C 3 N 4 electrocatalyst (Fig. 5c ) still exhibits a higher HER activity than the CO 2 reduction activity, but the amount of CO is much larger than for the MoS 2 -CDots-C 3 N 4 catalyst (the FE of CO production reaches 25%, inset of Fig. 5c ). It can be thus concluded that the concept of the ternary HER-CDots-C 3 N 4 is general and valid for HER catalysts different than Co 3 O 4 . Achievement of a relatively high amount of CO/H 2 however requires the application of a HER catalyst with only a medium activity pushing the balance between HER and CO 2 reduction toward CO 2 reduction. The smaller the HER activity, the larger relative amount of CO is obtainable. This conclusion was directly checked by reducing the amount of Au in the ternary Au-CDots-C 3 N 4 electrocatalyst. The electrochemical tests (Fig. 5d ) show that decreasing the amount of Au by a factor of two enabled the generation of syngas with a CO to H 2 volume ratio larger than one. A striking property of the h-Au-CDots-C 3 N 4 catalyst is its extremely high mass activity for producing syngas, i.e., >700 A/g Au for CO production and >700 A/g Au H 2 production (~1500 A/g Au for the total current) at −0.7 V for the catalyst shown in Fig. 5d . This activity is two orders of magnitude larger than previously reported for efficient Au electrodes for CO production [17] , [18] . This high mass activity allows a reduction of the electrode cost when precious catalysts (e.g., Au) are applied. Fig. 5 Catalytic activity of composite catalysts with different HER catalysts. a Current density for HER ( j H2 , black trace) vs. the applied potential, catalyzed by Pt-CDots-C 3 N 4 in CO 2 -saturated 0.5 M KHCO 3 electrolyte. b Current density for HER ( j H2 , black trace) and current density for CO 2 reduction to CO, ( j co , red trace) and FEs of H 2 and CO (inset) vs. the applied potential, catalyzed by MoS 2 -CDots-C 3 N 4 in CO 2 -saturated 0.5 M KHCO 3 electrolyte. c Current density for HER ( j H2 , black trace) and current density for CO 2 reduction, ( j co , red trace) and FEs of H 2 and CO (inset) vs. the applied potential, catalyzed by Au-CDots-C 3 N 4 in CO 2 -saturated 0.5 M KHCO 3 electrolyte. d Current density for HER ( j H2 , black trace) and current density for CO 2 reduction, ( j co , red trace) and FEs of H 2 and CO (inset) vs. the applied potential, catalyzed by Au-CDots-C 3 N 4 in CO 2 -saturated 0.5 M KHCO 3 electrolyte. The amount of Au in d is half of that in c (marked as h-Au-CDots-C 3 N 4 ) leading to an increase of the CO/H 2 ratio in d with respect to that in c Full size image The design concept of the HER-CDots-C 3 N 4 EC catalyst for syngas generation was introduced and its electrocatalytic performance for syngas production in aqueous solutions was studied, applying Co 3 O 4 , MoS 2 , Au, and Pt as the HER catalyst component. The Co 3 O 4 -CDots-C 3 N 4 electrocatalyst was found the most efficient for syngas production among the composite combinations investigated. The Co 3 O 4 -CDots-C 3 N 4 is capable of controlling the balance between the HER channel and CO 2 reduction channel. The Co 3 O 4 -CDots-C 3 N 4 initiates the reaction of CO 2 reduction to CO in aqueous solutions at a low overpotential (0.17 V) while the total current density reaches up to 15 mA/cm 2 at a potential of −1.0 V. The mass activity of the Co 3 O 4 -CDots-C 3 N 4 is ~10 A/g catalyst at −0.6 V when the total mass of the catalyst is considered and 1–2 orders of magnitude larger when the mass of the HER catalyst is considered (which is ~0.5–5% of that of the total catalyst weight). The Co 3 O 4 -CDots-C 3 N 4 induces high FEs (95%) and is characterized by a stable production of syngas (over 100 h). Notably, the H 2 /CO ratio of syngas produced applying Co 3 O 4 -CDots-C 3 N 4 is tunable from 0.07:1 to 4:1 by controlling the applied potential. The H 2 /CO may be also tuned by varying the amount of Co 3 O 4 in the Co 3 O 4 -CDots-C 3 N 4 . Dedicated experiments validated the catalyst design concept and provided additional insight to the syngas generation processes. C 3 N 4 and Co 3 O 4 are the activity sites for CO 2 reduction reaction and HER, respectively. CDots are the generation site of H• needed to trigger both the reduction of CO 2 to CO and the HER. The three-component catalyst concept is a general one and may be applied to a host of other materials. The versatility of the three components composite design may open a powerful pathway for the development of high-performance catalysts for syngas production as well as for other chemicals generation. Such an efficient and cost-effective electrocatalytic system has a high potential to be employed for the large-scaled production of syngas and controlled mixtures of other chemicals from CO 2 . Instruments Transmission electron microscopy (TEM), high-resolution transmission electron microscopy (HRTEM), and scanning TEM (STEM) images were obtained using a FEI/Philips Tecnai G2 F20 TWIN transmission electron microscope. The energy dispersive X-ray spectroscopy (EDS) analyses were taken on a FEI-quanta 200 scanning electron microscope with an acceleration voltage of 20 kV. The crystal structure of the resultant products was characterized by X-ray diffraction (XRD) using an X’Pert-ProMPD (Holland) D/max-γAX-ray diffractometer with Cu Kα radiation ( λ = 0.154178 nm). X-ray photoelectron spectroscopy (XPS) was obtained by using a KRATOS Axis ultra-DLD X-ray photoelectron spectrometer with a monochromatized Mg Kα X-ray source ( hν = 1283.3 eV). The electrocatalysis reactions were tested by a Model CHI 660C workstation (CH Instruments, Chenhua, Shanghai, China). The electrochemical impedance spectroscopy (EIS) measurements were obtained applying a CHI 832 electrochemical instrument (CHI Inc., USA). Materials KHCO 3 (99.7%) and Nafion perfluorinated resin solution (5 wt.%) were purchased from Sigma-Aldrich; hydrogen (99.999%), nitrogen (99.999%), and carbon dioxide (99.999%) were purchased from Airgas; Nafion®212 membrane was purchased from Dupont; Toray Carbon Paper (TGP-H-60) was purchased from Alfa Aesar; All chemicals were purchased from Sigma-Aldrich unless specifically stated. Milli-Q ultrapure water (Millipore, ≥18 MΩ/cm) was used throughout the work. Fabrication of electrocatalysts CDots were synthesized by our previously reported electrochemical etching method [34] . After 30-days reaction, a dark yellow solution containing CDots was formed in the reaction cell. It was then purified and concentrated to form a CDots solution of 3 mg/mL. For C 3 N 4 fabrication, 10 g of melamine powder was put into an alumina crucible with a cover and then heated to 550 °C at a rate of 0.5 °C per min in a muffle furnace and maintained at this temperature for 3 h. The yellow powder (C 3 N 4 ) was obtained after cooling down to room temperature. Co 3 O 4 NPs was synthesized by hydrothermal method. Twenty mL Co(NO 3 ) 2 (0.01 M) solution was added into an alumina crucible with a cover and then heated to 550 °C at a rate of 0.5 °C per min in a muffle furnace and maintained at this temperature for 3 h. The black powder (Co 3 O 4 NPs) was obtained after cooling down to room temperature. For preparation of Co 3 O 4 -C 3 N 4 , CDots-C 3 N 4 or Co 3 O 4 -CDots-C 3 N 4 , 10 g of melamine powder was mixed with 10 mL solution containing 0.05 M Co(NO 3 ) 2 , CDots, CDots and 0.05 M Co(NO 3 ) 2 , respectively. Then, the mixture was put into an alumina crucible with a cover and heated to 550 °C at a rate of 0.5 °C per min in a muffle furnace and maintained at this temperature for 3 h. For preparation of Co 3 O 4 -CDots, 10 mL solution containing 0.05 M Co(NO 3 ) 2 and CDots (3 mg/mL) was put into an alumina crucible with a cover and heated to 550 °C at a rate of 0.5 °C per min in a muffle furnace and maintained at this temperature for 3 h. Synthesis of Pt-CDots-C 3 N 4 An aliquot of 0.3 g CDots-C 3 N 4 (obtained by heating melamine at 550 °C for 3 h) was added into 10 mL H 2 PtCl 6 (2 mM) aqueous solution and stirred for 12 h. After centrifuging, the precipitate was irradiated by UV light for 10 h. The resulting product was collected by centrifugation and dried in a vacuum at 60 °C for 12 h. Synthesis of MoS 2 -CDots-C 3 N 4 An aliquot of 0.3 g CDots-C 3 N 4 (obtained by heating melamine at 550 °C for 3 h) was added into 15 mL aqueous solution containing Na 2 MoO 4 (0.0625 g) and L-cysteine (0.1 g). The mixed solution was stirred 3 min. After that, the mixture was poured into a Teflon-lined stainless steel autoclave, and heated at 180 °C for 24 h. After the autoclave was cooled down to room temperature, the resulting black sediments were collected by centrifugation (10,000 rpm, 10 min) and washed with deionized water and ethanol for several times, and then dried in a vacuum oven at 80 °C for 12 h [37] . Synthesis of Au-CDots-C 3 N 4 and h-Au-CDots-C 3 N 4 An aliquot of 0.3 g CDots-C 3 N 4 (obtained by heating melamine at 550 °C for 3 h) was added into 10 mL HAuCl 4 (2 mM or 1 mM) aqueous solution and stirred for 12 h. After centrifuging, the precipitate was irradiated by UV light for 2 h. The resulting product was collected by centrifugation and dried in vacuum at 60 °C for 12 h [38] . Electrocatalysis activity test Electrocatalysis activity test experiments were performed using a standard three-electrode configuration. A platinum wire was used as an auxiliary electrode and a saturated calomel electrode (SCE) was used as a reference electrode. The working electrode was either a catalyst-modified carbon fiber paper electrode (CFPE for short, 0.7 cm × 0.7 cm), or a catalyst-modified glassy carbon disk electrode (GCE for short, 3.0 mm diameter). For product analysis and constant-potential electrolysis experiment, the CFPE working electrode was a catalyst-modified carbon fiber paper electrode (0.7 cm × 0.7 cm). The preparation of the CFPE working electrode is as follows. An aliquot of 1.3 mg of electrocatalyst was ground with 0.1 mg polyvinylidene fluoride (PVDF) with a few drops of 1-methyl-2-pyrrolidone (MP) added to the produced mixture. The mixture was added into 10 mL 0.5% Nafion solution. After sonication, 1 mL dispersed solution was dropped directly onto the two sides of a 0.7 cm × 0.7 cm carbon fiber paper (the two sides of the carbon paper were modified by the catalyst). The bulk electrolysis was performed in an airtight electrochemical H-type cell with three electrodes. H-type cell consists of two compartments (volume of each part is 115 mL) separated by a Nafion®212 anion exchange membrane with 75 mL 0.5 M KHCO 3 electrolyte in each chamber and. Besides, LSV experiments were used with the catalyst-modified GCE as the working electrode. The preparation of the GCE working electrode is as follows. 6 mg electrocatalyst was added into 2 mL 0.5% Nafion solution. After sonication, 3 μL dispersed solution was dropped on GCE. The mass density of catalyst was 0.127 mg/cm 2 . The electrochemical tests of different catalysts combinations were performed with full loading, i.e., the mass of the composite catalyst was 9 µg (Supplementary Table 4 ). The electrochemical surface area (ECSA) test of single catalyst components were performed using partial loading, i.e., 1% of 9 µg CDots and 6% of 9 µg Co 3 O 4 (Supplementary Table 4 ). For LSVs experiments, initially, polarization curves for the modified electrode were carried out under an inert N 2 (gas) atmosphere. After this, the solution was purged with CO 2 (99.999%) for at least 30 min (CO 2 -saturated high purity aqueous 0.5 M KHCO 3 ) and the electrocatalytic CO 2 reduction was measured. Data availability The data that support the findings of this study within the paper and its Supplementary Information file are available from the corresponding authors on request.